Lfng regulates the synchronized oscillation of the mouse segmentation clock viatrans-repression of Notch signalling The synchronized oscillation of segmentation clock is required to generate a sharp somite boundary during somitogenesis. However, the molecular mechanism underlying this synchronization in the mouse embryos is not clarified yet. We used both experimental and theoretical approaches to address this key question. Here we show, using chimeric embryos composed of wild-type cells and Delta like 1 ( Dll1 )-null cells, that Dll1-mediated Notch signalling is responsible for the synchronization mechanism. By analysing Lunatic fringe ( Lfng ) chimeric embryos and Notch signal reporter assays using a co-culture system, we further find that Lfng represses Notch activity in neighbouring cells by modulating Dll1 function. Finally, numerical simulations confirm that the repressive effect of Lfng against Notch activities in neighbouring cells can sufficiently explain the synchronization in vivo . Collectively, we provide a new model in which Lfng has a crucial role in intercellular coupling of the segmentation clock through a trans -repression mechanism. The metameric features of vertebrates are based on the structure of the somites, which are sequentially produced (one by one) as a segmented cell mass from the anterior end of the presomitic mesoderm (PSM). The timing of this periodicity is controlled by the oscillation of gene expression, so called segmentation clock [1] . In mice, the core component of the segmentation clock is the negative feedback loop that regulates Hes7 expression and incorporates another clock gene Lunatic fringe ( Lfng ), the product of which in turn represses Notch activation and generates Notch signal activity oscillations [2] , [3] , [4] , [5] . In addition, a synchronization mechanism is required to form a sharp somite boundary [6] , [7] , [8] . Although the intracellular mechanisms that underlie the activities of these oscillators are now well understood [9] , the regulation of the intercellular coupling among clock cells that enable synchronization is largely unknown in mice [10] . In zebrafish somitogenesis, a Notch signalling-mediated coupled oscillator model has been proposed, in which the oscillation of Her1 and Her7 (orthologues of mouse Hes7) is synchronized between neighbouring cells via the function of DeltaC oscillation under the control of Her1/7 (refs 11 , 12 ). In the mouse, however, the issues of whether Notch signals are essential for the synchronization of the segmentation clock and how this event is regulated, have remained elusive. Notch signalling is required for the induction of several genes including clock genes, thus it has been difficult to analyse synchronization mechanisms independent of gene expression regulation. Here we adopted chimera analyses to overcome this difficulty and clarified that Notch signalling is required not only for the oscillation of the mouse segmentation clock, but also for its synchronization. In addition, we propose that Lfng has an important role in the synchronization mechanism via both chimera experiments and numerical simulation. Notch signalling synchronizes the segmentation clock To examine the involvement of Notch signal in the clock synchronization mechanism during mouse somitogenesis, we established a method to quantify the rate of synchronization based on the Hes7 protein expression levels and on the amount of cleaved Notch1 receptor ( Fig. 1a,b ; Supplementary Figs S1, S2 ). We defined relative PSM position as 0–100% from the anterior to posterior PSM, and defined the posterior PSM region as 30–100% to avoid Mesp2-expressing domain (anterior PSM). The rate of synchronization is calculated at an anterior part of the posterior PSM, as the regulation of gene expression changes once Mesp2 is expressed [5] , [13] , [14] , and gene expression mainly depends on FGF signalling in the posterior part of the posterior PSM [15] . Therefore, we focused on the narrow PSM region (30–34%), where we can observe the outcome of synchronized expression of segmentation clock genes clearly. In the wild-type embryos, the synchronization rates for Hes7 and Notch activity were 77±6% and 86±8%, respectively ( Fig. 1c–e ). Next, we analysed Dll1 -knockout (KO) embryos, which are defective in activating Notch signalling [16] , and Lfng -KO embryo, which are defective in repressing Notch signalling [5] . In Dll1 -KO embryo, however, Hes7 expression was too low to determine the synchronization rate although Hes7 still oscillated in the posterior part of the PSM ( Fig. 1f ). In Lfng -KO embryo, Hes7 expression oscillated in the anterior region of the posterior PSM and the synchronization rate was calculated as 53±3% ( Fig. 1g ). However, we judged the Lfng -null embryos as an inappropriate system to examine synchronization, as we cannot distinguish whether the defect is due to the defect in the synchronization mechanism or in the clock system by the constitutive activation of Notch signalling. Hence, we needed to develop a system in which the intracellular segmentation clock mechanism is intact but which shows impaired intercellular coupling because of the partial inhibition of Notch/Delta signalling. 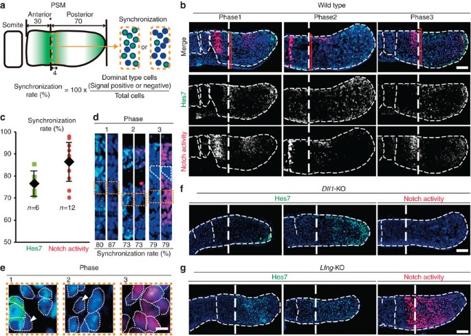Figure 1: Methods used to calculate the synchronization rate of the mouse segmentation clock. (a) The Hes7 and Notch activity levels were analysed at the defined PSM region, which was separated into two parts, anterior and posterior. The synchronization rate was then calculated at the 30–34% area of the PSM using the formula shown. (b) Segmentation clock patterns of three distinct phases in the wild-type mouse embryo visualized by analysing the Hes7 (green) and Notch activity (red) levels along the anterior–posterior axis in the posterior PSM. Blue indicates nuclei. Thin white dotted lines represent the somite and PSM. Thick white dotted lines indicate the anterior limit of the posterior PSM. (c) Synchronization rates of wild-type mouse embryos calculated by detecting the Hes7 (green square) or Notch activity (red circle) levels are shown. Error bars represent s.d. (d) Magnified images at the 30–34% the PSM ofb(indicated by red strips) were used to calculate synchronization rate shown inc. Hes7 (left) and Notch activity (right) for each phase, exhibiting the reverse phase are shown. Non-PSM cells indicated by white dotted lines were excluded from these calculations. (e) Magnified images of the areas enclosed by the brown dotted lines ind. White triangles indicate de-synchronized cells. (f,g) The Hes7 expression (green) and Notch activity (red) patterns inDll1-KO andLfng-KO embryos. There is no Notch activity in theDll1-KO embryo, whereas all cells show Notch activity in theLfng-KO embryo. Scale bars, 100 μm (b,f,g), 10 μm (e). In images, non-specific signals due to blood cells were removed. Figure 1: Methods used to calculate the synchronization rate of the mouse segmentation clock. ( a ) The Hes7 and Notch activity levels were analysed at the defined PSM region, which was separated into two parts, anterior and posterior. The synchronization rate was then calculated at the 30–34% area of the PSM using the formula shown. ( b ) Segmentation clock patterns of three distinct phases in the wild-type mouse embryo visualized by analysing the Hes7 (green) and Notch activity (red) levels along the anterior–posterior axis in the posterior PSM. Blue indicates nuclei. Thin white dotted lines represent the somite and PSM. Thick white dotted lines indicate the anterior limit of the posterior PSM. ( c ) Synchronization rates of wild-type mouse embryos calculated by detecting the Hes7 (green square) or Notch activity (red circle) levels are shown. Error bars represent s.d. ( d ) Magnified images at the 30–34% the PSM of b (indicated by red strips) were used to calculate synchronization rate shown in c . Hes7 (left) and Notch activity (right) for each phase, exhibiting the reverse phase are shown. Non-PSM cells indicated by white dotted lines were excluded from these calculations. ( e ) Magnified images of the areas enclosed by the brown dotted lines in d . White triangles indicate de-synchronized cells. ( f , g ) The Hes7 expression (green) and Notch activity (red) patterns in Dll1 -KO and Lfng -KO embryos. There is no Notch activity in the Dll1 -KO embryo, whereas all cells show Notch activity in the Lfng -KO embryo. Scale bars, 100 μm ( b , f , g ), 10 μm ( e ). In images, non-specific signals due to blood cells were removed. Full size image To make this condition, we thus generated a Dll1 chimera composed of wild-type cells genetically marked with GFP and Dll1 -null cells ( Fig. 2a ; Supplementary Fig. S3a,c ). We assumed that if a cell in this embryo came into contact with at least one wild-type (Dll1-active) cell, the oscillation of the clock would recover as even Dll1 -null cells harbour Notch receptors and can therefore receive and process the Notch signals required for the proper oscillation of Hes7 (refs 15 , 17 ) ( Fig. 2b ). Under these conditions, if Notch signalling is essential only for oscillation but not for clock synchronization, we expect to observe the synchronization of oscillation in this Dll1 chimera. In contrast, if Notch signalling is required for synchronization, this is expected to be impaired in the Dll1 chimera. Our analyses indicated the latter to be the case. We first confirmed that there was a random distribution of Dll1 -null cells in this chimeric embryo and that wild-type cells, although present at very low levels, were often found in the vicinity of the Dll1 -null cells, indicating that most cells could receive a Notch signalling ( Supplementary Fig. S4 ). The segmentation clock oscillated even in Dll1 -null cells in this chimeric embryo, as revealed by different transcriptional states of Lfng , a sensitive clock marker ( Supplementary Fig. S5a–f, m–r ) [17] , [18] . However, the synchronization of the clock was found to be severely impaired in Dll1 chimera when the contribution rate of wild-type cells was low; Hes7 expression and Notch activity did not show a clear segregation pattern in the posterior PSM unlike in wild-type or chimeric embryo with high contribution rate of wild-type cells ( Fig. 2c ). The quantified synchronization rates were low in the chimeras with a low number of wild-type cells ( Fig. 2d,e , Supplementary Table S1 ). These results indicate that Dll1-mediated Notch signalling has a crucial role not only in clock oscillation but also in its synchronization during mouse somitogenesis. 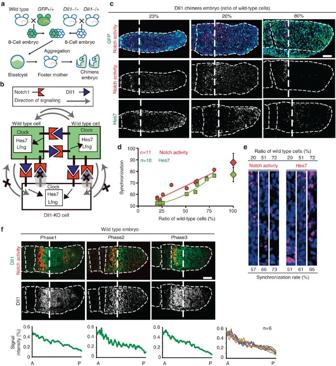Figure 2: Notch signalling regulates the segmentation clock during mouse somitogenesis. (a) Schematic representation of the procedure used to generate chimeric mouse embryos. Wild-type cells can be distinguished fromDll1-null cells by detecting EGFP signals. (b) A working hypothesis for how the synchronization mechanism can operate in a Dll1 chimeric embryo. Both wild-type cells andDll1-null cells will have functional clock systems and all will have the capacity to receive Notch signals from neighbouring wild-type cells. However, Notch signals cannot be transmitted byDll1-null cells. (c) The segmentation clock pattern in Dll1 chimeric embryos. Neither the Notch activity nor Hes7 expression levels showed a clear segregation pattern in the posterior PSM with low contribution rate of wild-type cells. In images, non-specific signals were removed. (d) The synchronization rate of a Dll1 chimeric embryo measured through the Notch activity (red circle) and Hes7 expression (green square) profiles. Diamonds indicate the synchronization rate in the wild-type embryos. Error bars represent s.d. (e) Notch activity and Hes7 expression patterns in the 30–34% area of the posterior PSM. Upper numbers indicate the contribution rates of wild-type cells in each chimera and lower numbers indicate the synchronization rates. (f) Dll1 protein expression at each segmentation clock phase (judged using the Notch activity pattern, red). Dll1 expression (green) was detectable in almost similar patterns using a Dll1 N-terminus antibody. Graphs indicate the signal intensity of the Dll1 protein expression in the posterior PSM of each upper image; the right-most figure is a merged graph of the Dll1 protein expression data (n=6). Scale bars, 100 μm. Figure 2: Notch signalling regulates the segmentation clock during mouse somitogenesis. ( a ) Schematic representation of the procedure used to generate chimeric mouse embryos. Wild-type cells can be distinguished from Dll1 -null cells by detecting EGFP signals. ( b ) A working hypothesis for how the synchronization mechanism can operate in a Dll1 chimeric embryo. Both wild-type cells and Dll1 -null cells will have functional clock systems and all will have the capacity to receive Notch signals from neighbouring wild-type cells. However, Notch signals cannot be transmitted by Dll1 -null cells. ( c ) The segmentation clock pattern in Dll1 chimeric embryos. Neither the Notch activity nor Hes7 expression levels showed a clear segregation pattern in the posterior PSM with low contribution rate of wild-type cells. In images, non-specific signals were removed. ( d ) The synchronization rate of a Dll1 chimeric embryo measured through the Notch activity (red circle) and Hes7 expression (green square) profiles. Diamonds indicate the synchronization rate in the wild-type embryos. Error bars represent s.d. ( e ) Notch activity and Hes7 expression patterns in the 30–34% area of the posterior PSM. Upper numbers indicate the contribution rates of wild-type cells in each chimera and lower numbers indicate the synchronization rates. ( f ) Dll1 protein expression at each segmentation clock phase (judged using the Notch activity pattern, red). Dll1 expression (green) was detectable in almost similar patterns using a Dll1 N-terminus antibody. Graphs indicate the signal intensity of the Dll1 protein expression in the posterior PSM of each upper image; the right-most figure is a merged graph of the Dll1 protein expression data ( n =6). Scale bars, 100 μm. Full size image The expression of Dll1 does not oscillate in the mouse PSM In zebrafish somitogenesis, the intercellular coupling of the clock cells that are essential for synchronization is achieved through the cyclic expression of DeltaC under the control of Her1 and Her7 oscillation [11] , [12] , [19] , [20] . To determine whether a similar mechanism is responsible for intercellular coupling in mice, we examined the protein expression of Dll1 at different clock phases by immunostaining. Although the Dll1 protein signals displayed a high-to-low gradation along the A–P axis, the expression pattern was uniform at all clock phases. This indicates that Dll1 does not show clear protein oscillation during mouse somitogenesis, at least at E10.5, which is consistent with a previous report on Dll1 mRNA expression ( Fig. 2f ) [13] . Hence, unlike the situation in zebrafish, intercellular coupling is unlikely to be regulated in the mouse through the control of the Dll1 gene. Lfng represses Notch signalling in the neighbouring cells We next focused on the Lfng gene as an appropriate candidate gene for the regulator of the clock synchronization in the mouse, as Lfng oscillates and has an important role in the mouse [5] , [17] but not in the zebrafish embryo [21] . Lfng is a glycosyltransferase known to both positively [22] , [23] and negatively [4] , [5] , [17] modulate Notch activity via the glycosylation of the Notch receptor in a cell-autonomous manner. However, it is not known whether Lfng also regulates Notch signalling in neighbouring cell. We speculated that Lfng might influence the intercellular coupling of the segmentation clock if it has the ability to affect Notch activity in neighbouring cells by modulating Dll1 function in the same cell. To test this attractive possibility, we generated a chimeric embryo composed of wild-type and Lfng-null cells ( Fig. 3a ; Supplementary Fig. S3b,c ). As shown previously, Notch activity was elevated in all PSM cells in this Lfng -KO embryo ( Figs 1g , 3b ). In the chimera embryo, wild-type cells exhibit a positive or negative signal for Notch activity. Interestingly, however, a positive or negative signal was also observed in the Lfng -null cells of the chimeric embryo ( Fig. 3b ), indicating that the Notch activity was being repressed by the function of Lfng expressed in the surrounding wild-type cells. 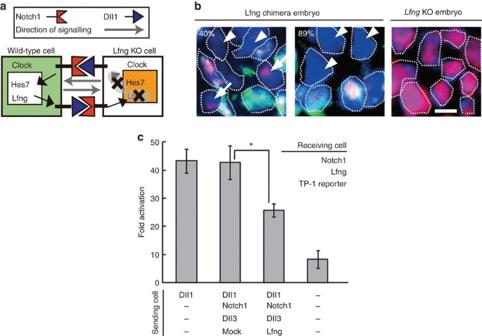Figure 3: Lfng represses Notch signalling in neighbouring cells via Dll1 function. (a) A working hypothesis for the intercellular coupling mechanism operating in the Lfng chimeric embryo. All PSM cells in this chimera can communicate with neighbouring cells by both sending and receiving Notch signalling. If Lfng modulates Notch activity in neighbouring cells, this activity inLfng-null cells may be affected by wild-type cells. (b) Notch activity (red) showing an ON (arrows) and OFF (arrowheads) state in theLfng-null cells of Lfng chimeric embryos. In contrast, Notch activity is always ON in theLfng-KO embryo. Green indicates wild-type cells and blue indicates nuclei. Scale bars, 10 μm. (c) Lfng repressed a signal-sending ability in NIH-3T3 cells expressing Dll1, Notch1 and Dll3 together with Lfng. Notch activity was assayed by TP-1-Luc-reporter activity included in the NIH-3T3-expressing Notch1 and Lfng (receiving) cells. The relative induction of luciferase activity in each sample was calculated and described as fold activation against the internal control. Error bars indicate s.d. of the mean from three experiments (*P<0.001, unpaired Student'st-test). Figure 3: Lfng represses Notch signalling in neighbouring cells via Dll1 function. ( a ) A working hypothesis for the intercellular coupling mechanism operating in the Lfng chimeric embryo. All PSM cells in this chimera can communicate with neighbouring cells by both sending and receiving Notch signalling. If Lfng modulates Notch activity in neighbouring cells, this activity in Lfng -null cells may be affected by wild-type cells. ( b ) Notch activity (red) showing an ON (arrows) and OFF (arrowheads) state in the Lfng -null cells of Lfng chimeric embryos. In contrast, Notch activity is always ON in the Lfng -KO embryo. Green indicates wild-type cells and blue indicates nuclei. Scale bars, 10 μm. ( c ) Lfng repressed a signal-sending ability in NIH-3T3 cells expressing Dll1, Notch1 and Dll3 together with Lfng. Notch activity was assayed by TP-1-Luc-reporter activity included in the NIH-3T3-expressing Notch1 and Lfng (receiving) cells. The relative induction of luciferase activity in each sample was calculated and described as fold activation against the internal control. Error bars indicate s.d. of the mean from three experiments (* P <0.001, unpaired Student's t -test). Full size image To more directly ask whether the suppressive effect of Notch activity by Lfng is transferred from signalling cells, we performed Notch signalling reporter assays using two kinds of cultured cells, one type being receiving cells, which express Notch1 and the reporter, and the other type being sending cells, which express Dll1, Dll3 and Notch1. We tried to reproduce similar condition in NIH3T3 cells to those of PSM cells in vivo and tested whether the ability of signalling cells was influenced by Lfng. We found that the Notch-reporter activity in the receiving cells was decreased when the signal-sending cells expressed Lfng ( Fig. 3c ). The cells in PSM also express Dll1, Dll3, Notch1 and Lfng, therefore, it was suggested that Lfng suppresses signal-sending capacity of Dll1 in the presence of Dll3 and Notch1. These results indicate that Lfng inhibits Dll1 function of signal-sending cells in a cell-autonomous manner and thereby suppresses Notch activity in the neighbouring cells. Simulation confirms the role of Lfng for synchronization To examine the sufficiency of our suggested model for the synchronization of the mouse segmentation clock, we performed and evaluated a series of numerical simulations consisting of a two-dimensional (2D) cell array corresponding to the cross-section perpendicular to the anterior–posterior axis of the mouse PSM. Thus, the 2D array of the simulation corresponds to 1D cell array in the experimental image (for example, 30–34% area of PSM). In vivo , the cells in this section are expected to synchronize their segmentation clock. Each cell contains a gene expression network containing the Notch signalling and Hes7 transcription pathways, as modelled in previous studies in zebrafish but modified in our current analysis in accordance with the results of corresponding studies in mouse [12] , [19] , [20] . Unlike the previous models proposed in the zebrafish, we did not include the gene regulation of Dll1 under the control of Hes7, but assumed that Dll1 expression is constant based on our current experimental observations ( Fig. 2f ). In addition, we included Lfng in our proposed model (see Supplementary Methods ). To evaluate the effect of the hypothesized regulation of Notch signalling by Lfng in trans , we initially did not include the well-established cell-autonomous repression of Notch signalling by Lfng, but evaluated the effects of this mechanism in later simulations [4] , [5] . We also introduced random gene expression noise so that without cell–cell communication, the phases of the segmentation clock within the cell population was randomized. Using these simulations, we were able to demonstrate that if Lfng represses Notch signalling in neighbouring cells, the phase of the segmentation clock in the mouse cell population synchronizes ( Fig. 4a,b ; Supplementary Movie S1 , S2 ). Importantly, if the trans -regulation of the Notch signalling by Lfng was activation and not repression, synchronization was not observed and the phases of the clock among neighbouring cells were opposing in a manner similar to lateral inhibition. The consequence of the simulation is not due to the specific values of the parameters. Even though we change the values of parameters, we see synchronization as long as the condition (parameter values) allows oscillation of the segmentation clock ( Supplementary Fig. S6 ). In summary, therefore we demonstrated using computer simulation that the repression of neighbouring Notch signalling by Lfng, but not activation, is sufficient to synchronize the segmentation clocks in the mouse. 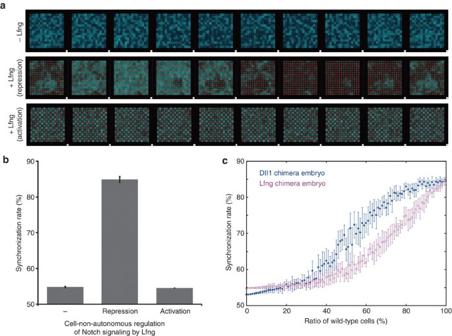Figure 4: Numerical simulation indicating thattrans-repression via Lfng is sufficient for clock synchronization. (a) Snapshots of the computer simulations. The phases of the segmentation clock in each cell in the 16×16 cell array are represented by blue shading (bright, high Hes7 protein; dark, low Hes7 protein). In the absence of Notch activity repression by Lfng in neighbouring cells ('−Lfng'), the clock phase in each cell is not synchronized due to random noise introduced during the simulation. Under these same conditions, however,trans-repression of Notch signalling by Lfng ('+Lfng (repression)') resulted in phase synchronization. Moreover, if thetrans-regulatory event was activation ('+Lfng (activation)') rather than repression, the phases of the neighbouring cells became opposite. (b) The synchronization rates were calculated withouttrans-regulation ('−') or with thetrans-repression ('repression') or -activation ('activation') of Notch signalling by Lfng. (c) Synchronization of the segmentation clock in simulated chimeric cell arrays. The synchronization rate of Hes7 is plotted against the chimera rate. Simulations were conducted with thetrans-repression of Notch signal by Lfng but with random mixtures ofDll1-null cells (the concentrations ofDll1mRNA and protein were set to zero, blue) orLfng-null cells (the concentrations ofLfngmRNA and protein were set to zero, magenta) with wild-type cells in various ratios (the ratios of wild-type cells are indicated on the horizontal axis). Error bars indicate s.d. among ten trials for each data point. Figure 4: Numerical simulation indicating that trans -repression via Lfng is sufficient for clock synchronization. ( a ) Snapshots of the computer simulations. The phases of the segmentation clock in each cell in the 16×16 cell array are represented by blue shading (bright, high Hes7 protein; dark, low Hes7 protein). In the absence of Notch activity repression by Lfng in neighbouring cells ('−Lfng'), the clock phase in each cell is not synchronized due to random noise introduced during the simulation. Under these same conditions, however, trans -repression of Notch signalling by Lfng ('+Lfng (repression)') resulted in phase synchronization. Moreover, if the trans -regulatory event was activation ('+Lfng (activation)') rather than repression, the phases of the neighbouring cells became opposite. ( b ) The synchronization rates were calculated without trans -regulation ('−') or with the trans -repression ('repression') or -activation ('activation') of Notch signalling by Lfng. ( c ) Synchronization of the segmentation clock in simulated chimeric cell arrays. The synchronization rate of Hes7 is plotted against the chimera rate. Simulations were conducted with the trans -repression of Notch signal by Lfng but with random mixtures of Dll1 -null cells (the concentrations of Dll1 mRNA and protein were set to zero, blue) or Lfng -null cells (the concentrations of Lfng mRNA and protein were set to zero, magenta) with wild-type cells in various ratios (the ratios of wild-type cells are indicated on the horizontal axis). Error bars indicate s.d. among ten trials for each data point. Full size image Prediction of chimera experiments by simulation We next predicted the consequences of chimerization in our mouse segmentation clock model. We simulated a Dll1 chimera or Lfng chimera through the introduction of Dll1 -null or Lfng -null cells, respectively, and scored the resulting synchronization data ( Fig. 4c ; Supplementary Figs S7–S9 ). Increases in the rate of the Dll1 -null or Lfng -null cells decreased the level of synchronization as expected. However, in the simulations, we noticed that the maximum cluster size of the cell array both quantitatively and theoretically accounts for the synchronization rate in the chimera ( Supplementary Fig. S7 ). The maximum cluster size is the maximum number of wild-type cells adjoining each other without being interrupted by mutant cells. Because both the Dll1 -null and Lfng -null cells are defective for transmitting the synchronization signal, the null cells act as a barrier against the synchronization among wild-type cell clusters. Hence, the maximum cluster size is expected theoretically to correlate with the synchronization rate, and we did see such a correlation in the simulation. Importantly, also the synchronization was found to be more sensitive to the inclusion of Lfng -null cells compared with Dll1 -null cells, as a low number of Lfng -null cells disrupted synchronization more severely ( Fig. 4c , magenta versus blue). This same result was obtained whether or not we included the cell-autonomous repression of Notch signalling by Lfng ( Fig. 4c ; Supplementary Figs S10–S12 ). In our current working model, Lfng -null cells send an elevated amount of Dll1 signal in a constitutive manner to the neighbouring cells, regardless of the state of oscillation inside the Lfng -null cells. On receiving this high Dll1 input, the Notch signalling pathways in the neighbouring cells will reach an almost saturated level that does not reflect the oscillation status of the neighbouring wild-type cells. Hence, Lfng -null cells not only block synchronization among wild-type cell clusters but also actively perturb the clock phases of neighbouring wild-type cells. In contrast, a Dll1 -null cell does not disrupt neighbouring wild-type cells due to the lack of signalling ability, but the Dll1 -null cell can receive Notch signal from neighbouring wild-type cells. Therefore, each of the synchronized cell clusters in the chimeric embryos should always be larger than the corresponding wild-type cell clusters in the Dll1 chimera and smaller in the Lfng chimera. This qualitative difference is reflected in the simulation results showing that the synchronization rate is always lower in the Lfng chimera than that in the Dll1 chimera with the same chimeric rate regardless of the model we used ( Supplementary Fig. S7c–f ). In conclusion, our simulation data predict that if our model is functioning in vivo , the inclusion of Lfng -null cells results in a more severe disruption of segmentation clock synchronization compared with the situation in Dll1 -null cells. Distinct consequences of Dll1 and Lfng chimera experiments To investigate whether we see distinct synchronization defect predicted by numerical simulation, we examined the synchronization rate in Lfng chimeric embryos with different contribution of wild-type cells ( Fig. 5a,b ). We first confirmed that the segmentation clock was functional in each cell by confirming the different transcriptional states of Hes7 and also that Dll1 expression did not change in the Lfng chimeric embryos ( Supplementary Figs S5g–l and S13 ) [17] , [18] . The simulation results predicted that the synchronization rate of the segmentation clock would be lower in the Lfng chimera than those in Dll1 chimeras with the same chimeric rate ( Fig. 4c ; Supplementary Figs S10–12 ). In fact, the synchronization rate of both Notch activity and Hes7 expression in the Lfng chimeric embryos showed more severe defects than those in the Dll1 chimeric embryos ( Fig. 5c,d ; Supplementary table S1 ). These results are consistent with the cluster size effect predicted by our simulations, indicating that our model for the synchronization mechanism of mouse segmentation clock is sufficient to account for the experimental results using the chimeric embryos. 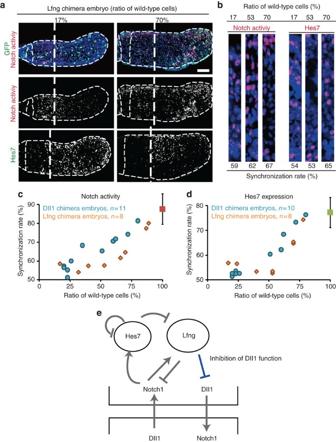Figure 5: Synchronization defects of Lfng and Dll1 chimeric embryos. (a) Segmentation clock pattern in Lfng chimeric embryos. Notch activity and Hes7 expression did not showed clear oscillation patterns. Scale bars, 100 μm. In images, non-specific signals were removed. (b) Notch activity and Hes7 expression patterns in the most anterior part of the posterior PSM. Upper numbers indicate the contribution rates of wild-type cells in each chimera and lower numbers indicate the synchronization rate. (c,d) The synchronization rate in the Lfng chimeric embryo (orange) compared with the Dll1 chimera (blue) measured using Notch activity (c) and Hes7 expression (d). Squares indicate the rate in wild-type embryos. Error bars represent s.d. (e) Our proposed model, in which Lfng regulates the intercellular coupling of Hes7 by inhibiting Dll1 function in addition to Notch1 activity. Figure 5: Synchronization defects of Lfng and Dll1 chimeric embryos. ( a ) Segmentation clock pattern in Lfng chimeric embryos. Notch activity and Hes7 expression did not showed clear oscillation patterns. Scale bars, 100 μm. In images, non-specific signals were removed. ( b ) Notch activity and Hes7 expression patterns in the most anterior part of the posterior PSM. Upper numbers indicate the contribution rates of wild-type cells in each chimera and lower numbers indicate the synchronization rate. ( c , d ) The synchronization rate in the Lfng chimeric embryo (orange) compared with the Dll1 chimera (blue) measured using Notch activity ( c ) and Hes7 expression ( d ). Squares indicate the rate in wild-type embryos. Error bars represent s.d. ( e ) Our proposed model, in which Lfng regulates the intercellular coupling of Hes7 by inhibiting Dll1 function in addition to Notch1 activity. Full size image In this study, we reveal that Notch signalling has a crucial role not only in the maintenance of clock oscillation but also in its synchronization. The synchronization mechanism is similar to that in zebrafish, which uses DeltaC-mediated coupled oscillator, and Dll1 is an important factor for synchronizationalso in mice. However, the regulation mechanism leading to the coupling of Notch activity is different in mice. Based on the results obtained from the chimera analysis, Notch signal reporter assays and the computer simulation, we propose that Lfng works cell autonomously to repress Dll1 function, thereby represses Notch signalling in neighbouring cells, and regulates the synchronized oscillation of Hes7 via intercellular coupling ( Fig. 5e ). In previous reports, Lfng is shown to enhance Notch signalling by promoting binding between ligands and Notch receptors in vivo [24] and in vitro [22] , [23] except in the PSM [4] , [5] , [17] . In ex vivo Notch signalling reporter experiments, we showed for the first time that Lfng inhibited Notch signalling in neighbouring cells. The molecular mechanism, in which Lfng inhibits Notch signalling in neighbouring cells, is an open question. A simplest scenario is that Lfng itself is secreted from a cell and affect Notch receptors in neighbouring cells. It is reported that Lfng has a secreted form [25] , however, our chimera analyses do not support the role of the secreted form in the synchronization mechanism. If the secreted form contributes to the synchronization mechanism independent of Dll1 function, we should have observed efficient clock synchronization even in the Lfng chimera in which the secreted Lfng can be supplied from wild-type cells. However, we did not observe such a phenomenon. Alternatively, our experiments collectively support that Lfng represses Dll1 function of the same cell and, consequently, represses Notch signalling in the neighbouring cells. Possible mechanisms of Lfng-dependent Dll1 repression includes the glycosylation modification of Dll1 by Lfng [26] or the modulation of Notch-Delta cis -interaction [27] by Lfng. Our reporter analyses indicated that trans -repression by Lfng was effective in the presence of Dll3 and Notch1 in signalling cells ( Fig. 3c ; Supplementary Fig. S14 ), suggesting that proper synchronization of segmentation clock may require Dll1, Dll3, Notch1 and Lfng. Further characterization of these components in both signal-sending and -receiving cells should be an important subject in the future studies. Animals and chimeric embryos The wild-type mice used in this study were MCH strain (Clea, Japan) genetically marked with CAG-EGFP [28] . The Dll1-lacZ knock-in [29] and Lfng KO mice [30] used for chimera production were provided by A. Gossler (Medizinische Hochschule Hannover, Hannover, Germany) and R. Johnson (University of Texas, Houston, USA). Dll1 +/flox ( Dll1-floxed-CAT-Dll3 knock-in) and Lfng +/Lfng−Venus ( Lfng-venus knock-in) mice were generated in our laboratory. Chimeric embryos were generated via the previously described aggregation method [31] . The details are provided in Supplementary Fig. S3 . Immunohistochemistry Following antigen retrieval, frozen sections (8 μm) were incubated with primary antibodies against cleaved Notch1 (1:200, Cell Signaling Technology), the Dll1 N-terminus [32] (G. Weinmaster) or the Dll1C-terminus [33] (K. Nakayama), followed by incubation with horseradish peroxidase-conjugated donkey anti-rabbit IgG antibody (1:200, Amersham Pharmacia Biotech) and Cyanin3-Tyramid detection reagent (Perkin-Elmer). GFP and Hes7 were detected using GFP antibodies (1:1,000, Abcam) or Hes7 (ref. 2 ; 1:100) antibodies, followed by incubation with an Alexa 488 donkey anti-chicken IgG (1:100, Molecular Probes) or Cyanin3-conjugated anti-guinea pig IgG (1:100, Abcam) secondary antibody, respectively. In situ hybridization and immunohistochemistry Following detection with anti-GFP antibodies, re-fixed sections were hybridized with digoxigenin-labelled anti-sense cRNA probes (Roche). The hybridized probes were detected using an horseradish peroxidase-conjugated anti-DIG sheep antibody (Roche) and Cyanin3-Tyramid (Perkin-Elmer) signal detection reagent. GFP was detected using an Alexa 488 donkey anti-chicken IgG secondary antibody (1:100, Molecular Probes). Method for calculation of the rate of synchronization After immunostaining with appropriate antibodies, we counted signal positive and negative cells using sections at 30–34% of PSM. We judged as positive if we find any signal above background in 4′,6-diamidino-2-phenylindole-positive nucleus ( Supplementary Fig. S2 ). The synchronization rate was calculated as dominant cell numbers (signal positive or negative)/total cell numbers (%) ( Fig. 1a ). Plasmids Complementary DNAs for murine Dll1 and Dll3 are kind gifts from S. Chiba (University of Tukuba, Ibaraki, Japan) and Sally L. Dunwoodie (Victor Chang Cardiac Research Institute, Australia), respectively. The cDNA of Lfng was originally cloned from cDNA of E14.5 fetal liver. All cDNA were cloned into the retrovirus vectors, Dll1 in pMY (gift from T. Kitamura, University of Tokyo, Tokyo, Japan), Dll3 in huko (gift from K. Hozumi, Tokai university, Isehara, Japan) and Lfng in ratCD2-expressing retrovirus vector MIGR (originally constructed by Hirano (Tokai University, Isehara, Japan)). NIH-3T3 cell lines used for the reporter assay To establish NIH-3T3 cell lines stably expressing Notch signalling components in various combinations, retroviruses encoding each molecule were obtained after transfection into the Plat-E ecotropic packaging cell line as described previously [34] . The integration of transfected genes was confirmed by detecting marker proteins linked by IRES (Dll1: GFP, Dll3: kusabira orange, Lfng: rat CD2 (detected by biotin-avidin system)). We used NIH3T3 and Notch1-expressing NIH3T3 as parental cell lines. Notch1-expressing NIH3T3 was established as a Zeosin-resistant stable transfectant with pTracer TM-CMV (Invitrogen, Carlsbad, CA) encoding mouse Notch1 , and Lfng was retrovirally transduced [35] . The transfectants were collected 48 h after the infection and the marker-positive cells were obtained by using a JSAN automatic cell sorter (Bay Bioscience, Kobe, Japan), giving rise to higher than 78.6% pure population as determined by post-sort analysis. Notch signalling reporter assay Reporter assays were carried out by the transient transfection of reporter plasmids TP1-luciferase ( pGa981-6 , including six copies of RBPJk-binding sites, constructed by L. Strobl [36] ) and pRL-TK (Promega, Madison, WI) into signal-receiving cell, Lfng-expressing Notch1/NIH3T3. This cell line was established from Notch1/3T3, a stable transfectant with pTracer TM-CMV (Invitrogen, Carlsbad, CA) encoding mouse Notch1 , and Lfng was retrovirally transduced. Reporter plasmids (0.38 mg) were co-transfected into 5×10 4 cells in 24-well plates by a liposome-based method (Lipofectamine LTX, Invitrogen) according to the manufacturer's instructions. Following 24 h culture after transfection, signal-receiving cells were detached by trypsinization and co-cultured with signal-sending cells (5×10 4 cells, respectively) for 40 h. After co-culture, cell lysates from the mixtures of two kinds of cells were then used for the luciferase assay using Dual luciferase reporter assay system (Promega, Madison, WI). Y.O. and Y.S. designed the research. Y.O. performed the in vivo experiments. N.A.-K. performed ex vivo experiments. T.S. and A.K. performed the mathematical modelling. Y.O., T.S., A.K. and Y.S. wrote the manuscript. J.K. and Y.S. supervised the project. How to cite this article: Okubo, Y. et al . Lfng regulates the synchronized oscillation of the mouse segmentation clock via trans -repression of Notch signalling. Nat. Commun. 3:1141 doi: 10.1038/ncomms2133 (2012).